Overproduction of stomatal lineage cells inArabidopsismutants defective in active DNA demethylation DNA methylation is a reversible epigenetic mark regulating genome stability and function in many eukaryotes. In Arabidopsis , active DNA demethylation depends on the function of the ROS1 subfamily of genes that encode 5-methylcytosine DNA glycosylases/lyases. ROS1-mediated DNA demethylation plays a critical role in the regulation of transgenes, transposable elements and some endogenous genes; however, there have been no reports of clear developmental phenotypes in ros1 mutant plants. Here we report that, in the ros1 mutant, the promoter region of the peptide ligand gene EPF2 is hypermethylated, which greatly reduces EPF2 expression and thereby leads to a phenotype of overproduction of stomatal lineage cells. EPF2 gene expression in ros1 is restored and the defective epidermal cell patterning is suppressed by mutations in genes in the RNA-directed DNA methylation pathway. Our results show that active DNA demethylation combats the activity of RNA-directed DNA methylation to influence the initiation of stomatal lineage cells. A network of genes that regulates stomatal development in Arabidopsis has been identified and established as a model for addressing fundamental questions such as how specific cell lineages are initiated and established, how stem cell-like asymmetric divisions are temporally maintained and how precursor cells ultimately differentiate into functional, mature structures [1] , [2] . Earlier studies have shown that three master bHLH genes, SPEECHLESS (SPCH) , MUTE and FAMA , act sequentially in stomatal fate transition and determination. The function of SPCH is especially important for the first step in the initiation of stomatal lineage cells [3] , [4] . Another important factor controlling the stomatal lineage cell population is EPIDERMAL PATTERNING FACTOR 2 ( EPF2 ). EPF2 belongs to a family of plant-specific, cysteine-rich peptides that is secreted by the early-stage lineage cells and acts as a negative regulator in stomata formation [5] , [6] . ROS1 is a bifunctional 5-methylcytosine DNA glycosylase/lyase critical for active DNA demethylation in most tissues of Arabidopsis plants [7] , [8] . ROS1 and its two paralogues, DEMETER-like 2 ( DML2 ) and DEMETER-like 3 ( DML3 ), are required for the prevention of DNA hypermethylation at thousands of genomic regions [9] , [10] , [11] . Loss-of-function mutations in these enzymes cause transcriptional silencing of some transgenes and endogenous genes [7] , [12] . Unlike another paralogue, DEMETER (DME), which is known to be critical for active DNA demethylation in the central cell and thereby for gene imprinting and endosperm development [13] , a developmental function has not been established for ROS1. In this study, we found that ROS1 loss-of-function mutants have a defect in epidermal cell patterning that is strikingly similar to the EPF2 loss-of-function phenotype. We further show that the promoter region of the EPF2 gene in ros1 mutants is hypermethylated, which leads to a dramatic decrease in its mRNA level. Our findings provide the first evidence that active DNA demethylation initiated by ROS1 plays an important role in controlling the dispersed stem cell population, the stomatal lineage cells, in plant development. ros1 mutant epidermis has more stomatal stem cells The loss-of-function mutants, ros1-4 and rdd ( ros1-3 dml2-1 dml3-1 ), do not exhibit apparent developmental phenotypes at the whole-plant level [11] . However, microscopic observation reveals that ros1-4 has clusters of small cells in the leaf epidermis, as exhibited in the epf2-1 mutant ( Fig. 1a–d and Supplementary Fig. 1 ). The ‘small-cell-cluster’ phenotype is more severe in the rdd triple mutant than in ros1-4 ( Fig. 1c,d and Supplementary Fig. 1 ); however, the ros1 mutation seems to be the major contributor to the phenotype in the rdd mutant. The number of small cells is more than three times greater in ros1-4 , rdd and rdd-2 ( ros1-4 dml2-2 dml3-2 ) than in the Col wild type, although the numbers of stomata are not different in the 3-day-old seedlings ( Fig. 1e ). Similar to ros1-4 , the ros1-3 and ros1-6 mutants also exhibit a ‘small-cell-cluster’ phenotype ( Supplementary Fig. 2 ). Furthermore, F1 progenies from ros1-4 × ros1-3 but not ros1-4 × Col or ros1-3 × Col display the mutant epidermal patterning phenotype ( Supplementary Fig. 3 ), and the phenotype in ros1-4 is largely rescued by expression of the wild-type ROS1 gene ( Fig. 2a–c ). Previous research showed that the clustered small cells in epf2 are stomatal lineage cells, which express the SPCH gene [6] . Because of the similarity in phenotypes, we suspected that the clustered, small cells in the ros1-4 epidermis could be stomatal lineage cells. We crossed the ros1-4 mutant with the stomatal cell fate-marker lines SPCHpro:nucGFP and MUTEpro:nucGFP . SPCH is required for the initiation of asymmetric cell division in stomatal development, and SPCHpro:nucGFP expression is mainly found in the early stomatal lineage cells [3] ( Fig. 3a ). As expected, all of the small-cell-clusters in ros1-4 have SPCHpro:nucGFP expression ( Fig. 3b,c ), demonstrating an enlarged population of stomata precursors in ros1 - 4 . In contrast, MUTE expression is required for termination of asymmetric cell division and it promotes the transition to guard mother cells (GMCs) [4] , and the expression of MUTEpro:nucGFP is restricted to the meristemoids in the wild-type Col ( Fig. 3d ). In ros1 - 4 , only a portion of the small-cell-clusters has MUTE expression ( Fig. 3e,f ). The behaviours of the SPCH and MUTE markers are consistent with those found in epf2 (ref. 6 ). We also examined the cotyledons of 10-day-old epf2-1 , ros1-4 , rdd and rdd-2 plants and found that these mutants have a similar increase in the numbers of stomata compared with the wild-type Col ( Supplementary Fig. 4 ). Together, these results suggest that some of the cells in the small-cell-clusters are arrested before the GMC stage in epf2-1 , ros1-4 , rdd and rdd-2 mutants. Therefore, similar to epf2 mutations ros1 mainly affects the specification of stomatal lineage cells but does not dramatically change the differentiation of these cells into GMC. 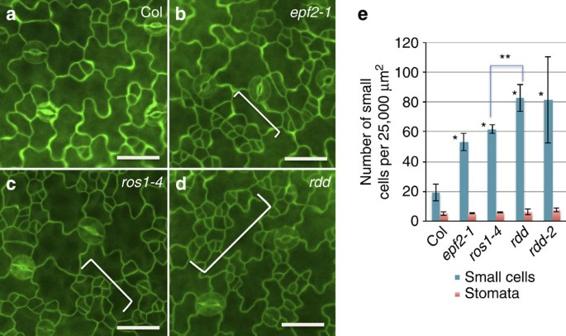Figure 1: Phenotypic analysis of epidermal patterning in theros1andrddmutants. (a–d) Microscopic image of cotyledon adaxial epidermal cells from 3-day-old Col (a),epf2-1(b),ros1-4(c) andrdd(d). Small-cell-clusters are indicated by brackets. (e) Numbers of clustered small cells and stomata for Col,epf2-1,ros1-4,rddandrdd-2. Values are means+s.d.’s per 25,000 μm2of 3-day-old cotyledon adaxial epidermis (n=3). Student’st-test, *P<0.03 (significantly different from Col), **P<0.02. Images ina–dare at the same magnification. Scale bar, 30 μm. Figure 1: Phenotypic analysis of epidermal patterning in the ros1 and rdd mutants. ( a – d ) Microscopic image of cotyledon adaxial epidermal cells from 3-day-old Col ( a ), epf2-1 ( b ), ros1-4 ( c ) and rdd ( d ). Small-cell-clusters are indicated by brackets. ( e ) Numbers of clustered small cells and stomata for Col, epf2-1 , ros1-4 , rdd and rdd-2 . Values are means+s.d.’s per 25,000 μm 2 of 3-day-old cotyledon adaxial epidermis ( n =3). Student’s t -test, * P <0.03 (significantly different from Col), ** P <0.02. Images in a – d are at the same magnification. Scale bar, 30 μm. 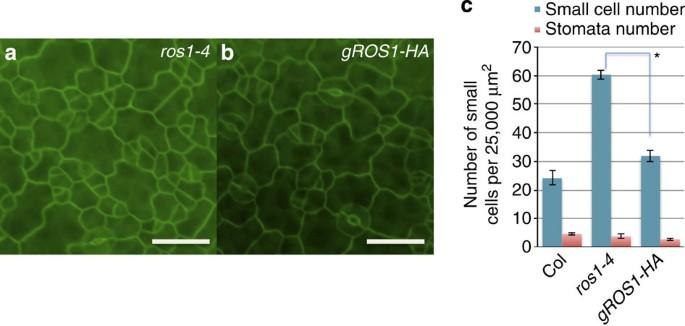Figure 2: Complementation analysis ofros1-4. Cotyledon epidermal cell phenotype of 3-day-old seedlings ofros1-π (a) andros1-4withgROS1-HA(b). The small-cell-cluster phenotype was rescued by expression of gROS1-HA. Scale bar, 30 μm. (c) Numbers of clustered small cells and stomata for Col,ros1-4,gROS1-HA. Values are means+s.d. per 25,000 μm2of 3-day-old cotyledon adaxial epidermis (n=3). Student’st-test, *P<0.02. Full size image Figure 2: Complementation analysis of ros1-4 . Cotyledon epidermal cell phenotype of 3-day-old seedlings of ros1 -π ( a ) and ros1-4 with gROS1-HA ( b ). The small-cell-cluster phenotype was rescued by expression of g ROS1 -HA. Scale bar, 30 μm. ( c ) Numbers of clustered small cells and stomata for Col, ros1-4 , gROS1-HA . Values are means+s.d. per 25,000 μm 2 of 3-day-old cotyledon adaxial epidermis ( n =3). Student’s t -test, * P <0.02. 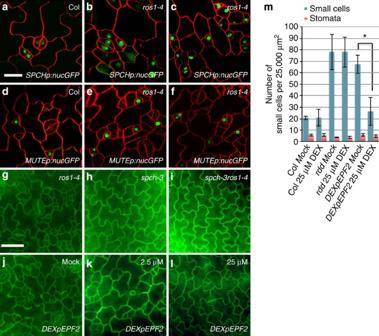Figure 3: Expression of stomatal lineage reporter genes inros1-4and genetic interactions betweenROS1,EPF2andSPCHin epidermal patterning. (a–f) Confocal images showing expression of the stomatal lineage reporter genesSPCHandMUTEin adaxial epidermal cells of 3-day-old Col andros1-4mutant seedlings.SPCHp:nucGFP(a–c),MUTEp:nucGFP(d–f). The genotypes are indicated above the images. Images ina–fare at the same magnification. Scale bar, 20 μm. (g–i) Genetic epistasis analysis ofspch-3andros1-4. (g)ros1-4, (h)spch-3and (i)ros1-4spch-3. (j–l) Modulation of the small-cell-cluster phenotype in therddmutant by expression of DEX-inducibleEPF2after treatment with (j) Mock (0 μM DEX), (k) 2.5 μM DEX and (l) 25 μM DEX. Images ing–lare at the same magnification. Scale bar, 30 μm. (m) Numbers of clustered small cells and stomata for Col,rddand therddmutant with DEX-inducibleEPF2 (DEXpEPF2)after treatment with Mock (0 μM DEX) or 25 μM DEX. Values are means+s.d.’s per 25,000 μm2of 3-day-old cotyledon adaxial epidermis (n=3). Student’st-test, *P<0.01. Full size image Figure 3: Expression of stomatal lineage reporter genes in ros1-4 and genetic interactions between ROS1 , EPF2 and SPCH in epidermal patterning. ( a – f ) Confocal images showing expression of the stomatal lineage reporter genes SPCH and MUTE in adaxial epidermal cells of 3-day-old Col and ros1-4 mutant seedlings. SPCHp:nucGFP ( a – c ), MUTEp:nucGFP ( d – f ). The genotypes are indicated above the images. Images in a – f are at the same magnification. Scale bar, 20 μm. ( g – i ) Genetic epistasis analysis of spch-3 and ros1-4 . ( g ) ros1-4 , ( h ) spch-3 and ( i ) ros1-4spch-3 . ( j – l ) Modulation of the small-cell-cluster phenotype in the rdd mutant by expression of DEX-inducible EPF2 after treatment with ( j ) Mock (0 μM DEX), ( k ) 2.5 μM DEX and ( l ) 25 μM DEX. Images in g – l are at the same magnification. Scale bar, 30 μm. ( m ) Numbers of clustered small cells and stomata for Col, rdd and the rdd mutant with DEX-inducible EPF2 (DEXpEPF2) after treatment with Mock (0 μM DEX) or 25 μM DEX. Values are means+s.d.’s per 25,000 μm 2 of 3-day-old cotyledon adaxial epidermis ( n =3). Student’s t -test, * P <0.01. Full size image ros1 mutations cause silencing of EPF2 Given the similarity in phenotypes of the ros1 and epf2 mutants, we next analysed the EPF2 expression level in ros1-4 , rdd and rdd - 2 mutants at the early seedling stage using quantitative RT–PCR. The results showed that EPF2 expression is dramatically reduced in the ros1-4 and rdd mutants relative to Col ( Fig. 4a ). As DNA methylation in promoter regions usually decreases gene transcription, we suspected that the reduced expression of EPF2 in ros1-4, rdd and rdd-2 might result from a hypermethylation of the EPF2 promoter DNA. We searched for the methylation status of the EPF2 promoter from the DNA methylomes of ros1-4 and rdd mutants [10] . The region upstream of the EPF2 promoter has an 835-bp hAT-like transposable element (TE) insertion with high methylation in Col, ros1-4 and rdd . We found increased DNA methylation levels in ros1-4 and rdd mutants relative to the wild-type Col in the EPF2 promoter immediately downstream of the TE insertion ( Fig. 4b ). Individual locus bisulfite sequencing confirmed that the EPF2 promoter is hypermethylated at all cytosine sequence contexts (CG, CHG and CHH, where H is C, A or T) in ros1-4 , rdd and rdd-2 ( Fig. 4c ). These results strongly suggested that DNA hypermethylation at the EPF2 promoter leads to the decreases in EPF2 expression that could be responsible for the small-cell-cluster phenotype in ros1-4 and rdd mutants. 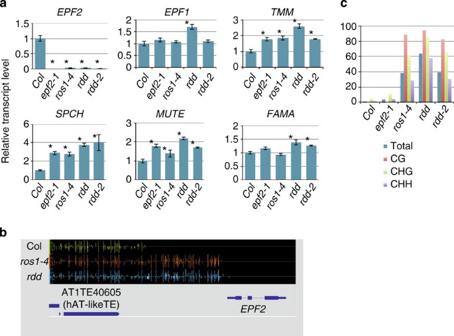Figure 4:EPF2expression and promoter DNA methylation. (a) Quantitative RT–PCR analysis of transcript levels ofEPF2and other stomata-related genes in 3-day-old Col,epf2-1,ros1-4,rddandrdd-2. Error bars represent s.d.’s (n=4). Student’st-test, *P<0.02 (significantly different from Col). (b) Snapshot in the Integrated Genome Browser showing DNA methylation levels of theEPF2promoter and upstream region in Col,ros1-4andrdd. (c) Bisulfite sequencing analysis of DNA methylation of theEPF2promoter in 3-day-old Col,epf2-1, ros1-4,rddandrdd-2. Figure 4: EPF2 expression and promoter DNA methylation. ( a ) Quantitative RT–PCR analysis of transcript levels of EPF2 and other stomata-related genes in 3-day-old Col, epf2-1 , ros1-4 , rdd and rdd-2 . Error bars represent s.d.’s ( n =4). Student’s t -test, * P <0.02 (significantly different from Col). ( b ) Snapshot in the Integrated Genome Browser showing DNA methylation levels of the EPF2 promoter and upstream region in Col, ros1-4 and rdd . ( c ) Bisulfite sequencing analysis of DNA methylation of the EPF2 promoter in 3-day-old Col, epf2-1, ros1-4 , rdd and rdd-2 . Full size image We also performed quantitative RT-PCR analysis for epf2-1 , ros1-4 , rdd and rdd-2 to measure changes in gene expression associated with stomatal development. The results indicated that, in epf2 , the genes involved in stomatal development, such as SPCH , MUTE , TMM , SCRM/ICE1 and ERL1 , are upregulated in expression relative to Col ( Fig. 4a and Supplementary Fig. 5 ). Consistent with the phenotypic similarity between epf2-1 and ros1-4 as revealed by microscopic observations, similar upregulation of these genes was also observed in ros1-4 , rdd and rdd-2 mutants ( Fig. 4a and Supplementary Fig. 5 ). The epidermal phenotype of ros1 is dependent on SPCH SPCH loss-of-function mutants lack stomata and have only jigsaw-puzzle-shaped pavement cells in their leaf epidermis [3] , [4] ( Fig. 3h ), which is nearly identical to those in EPF2 -overexpression lines [5] , [6] . Previous genetic and biochemical studies showed a tight connection between EPF2 and SPCH [14] . The perception of the EPF2 peptide by ERECTA is thought to activate a mitogen-activated protein kinase cascade that phosphorylates SPCH to downregulate its function [15] . Thus, EPF2 negatively regulates SPCH function at the early stage of stomatal development. If ROS1 regulates EPF2 expression and if the strong reduction in EPF2 gene expression is responsible for the small-cell-cluster phenotype in ros1-4 , we would expect the loss-of-function spch-3 mutation to be epistatic to ros1-4 . We crossed ros1-4 with spch-3 and generated ros1-4, spch-3 (−/−, +/−) plants. Of the progenies of selfed ros1-4, spch-3 (−/−, +/−) plants, 24.3% were of the ros1-4, spch-3 (−/−, −/−) genotype and showed the spch-3 phenotype ( Fig. 3g–i and Table 1 ). The genetic analysis indicates that ROS1 acts upstream of SPCH in stomatal development. Table 1 The segregation of the spch-3 mutant phenotype. Full size table EPF2 expression rescues the epidermal phenotype in rdd We next tested whether expression of EPF2 could rescue the small-cell-cluster phenotype in the rdd mutant. We generated rdd plants carrying the dexamethasone (DEX)-inducible EPF2 construct ( DEXpEPF2 ). The seedlings of DEXpEPF2 were germinated and grown on medium containing 2.5 or 25 μM DEX. The control plants grown on medium without DEX showed the rdd mutant phenotype ( Fig. 3j ). However, DEX-inducible ectopic expression of the EPF2 gene rescued the rdd mutant defect in epidermal cell patterning and small cell number ( Fig. 3j–m ). With a high concentration of DEX, part of the epidermis produced stomata-free or low-density area as previously observed when EPF2 was overexpressed [5] , [6] ( Fig. 3l ). These results clearly show that the reduced expression of EPF2 was responsible for the small-cell-cluster phenotype in ros1 and rdd mutants. EPF2 silencing and epidermal defect in ros1 depend on RdDM Previous work showed that the RD29Apro:luciferase transgene silencing triggered by ros1-1 can be suppressed by mutations in components of the RNA-directed DNA methylation (RdDM) pathway such as NUCLEAR RNA POLYMELASE D1 ( NRPD1 ) and HISTONE DEACETHYLASE6 ( HDA6 ) [16] . We constructed the double mutants nrpd1-3 ros1-4 and hda6 ros1-4 and used them to test whether the small-cell-cluster phenotype and EPF2 silencing and promoter DNA hypermethylation in ros1-4 are caused by RdDM. The nrpd1-3 and hda6 single mutants did not have significant epidermal defects ( Fig. 5a,c ). However, these mutations strongly suppressed the small-cell-cluster phenotype in the ros1-4 epidermis, since the epidermal patterning of nrpd1-3 ros1-4 and hda6 ros1-4 is almost identical to that of the nrpd1-3 or hda6 single mutants ( Fig. 5b,d,g ). The NRPD1 gene encodes the largest subunit of Pol IV, which is thought to act at an early step of the RdDM pathway leading to the biogenesis of 24-nt small interfering RNAs (siRNAs) that direct the de novo DNA methyltransferase DRM2 to methylate DNA at RdDM target loci ( Supplementary Fig. 6a ) [17] , [18] . Using small RNA northern blot analysis, we detected 24-nt siRNAs in ros1-4 as well as in Col with a probe from the EPF2 promoter ( Fig. 5j and Supplementary Fig. 7 ). The nrpd1 mutation blocked the accumulation of the siRNAs in Col and in the ros1-4 background ( Fig. 5j ). These results strongly suggest that the siRNAs are the initial trigger of EPF2 promoter DNA hypermethylation in ros1-4 . Furthermore, we crossed the DNA methyltransferase triple mutant drm1-2 drm2-2 cmt3-11 ( ddc ) and ros1-4 and constructed the drm1-2 drm2-2 cmt3-11 ros1-4 quadruple mutant and the drm1-2 cmt3-11 ros1-4 triple mutant. The epidermal patterns of drm1-2 drm2-2 cmt3-11 triple mutant were relatively normal ( Fig. 5e,g ). The drm1-2 cmt3-11 ros1-4 triple mutant still exhibited the small-cell-cluster phenotype; however, the phenotype was not observed in the drm1-2 drm2-2 cmt3-11 ros1-4 quadruple mutant ( Fig. 5f,g , Supplementary Fig. 6b,c ). The results indicated that the drm2-2 mutation was responsible for the suppression of the small-cell-cluster phenotype in the drm1-2 drm2-2 cmt3-11 ros1-4 quadruple mutant, which is consistent with DRM2 being the de novo methyltransferase in the RdDM pathway [17] , [18] . Consistent with microscopic observations, quantitative RT-PCR and bisulfite sequencing analyses showed that EPF2 expression levels and DNA methylation status at all cytosine contexts in the EPF2 promoter region in nrpd1-3 ros1-4 , ros1-4 hda6 and drm1-2 drm2-2 cmt3-11ros1-4 mutants were restored to almost the same level as in nrpd1 and hda6 single mutants or in the drm1-2 drm2-2 cmt3 - 11 triple mutant ( Fig. 5h,i ). Taken together, these results strongly suggest that siRNA-triggered de novo DNA methylation through the RdDM pathway is responsible for the DNA hypermethylation of the EPF2 promoter region and therefore for the downregulation of EPF2 gene expression in the ros1-4 mutant. 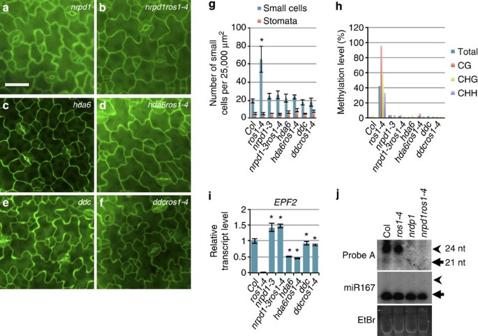Figure 5: Suppression of theros1epidermal patterning phenotype by RdDM mutations. (a–f) Adaxial epidermal cell phenotype of 3-day-old seedlings. (a)nrpd1-3, (b)nrpd1-3ros1-4, (c)hda6, (d)hda6ros1-4, (e)drm1-2drm2-2cmt3-13(ddc) and (f)drm1-2drm2-2cmt3-13ros1-4(ddcros1-4). Images ina–fare at the same magnification. Scale bar, 30 μm. (g) Numbers of clustered small cells and stomata for Col,ros1-4, nrpd1-3, nrpd1-3ros1-4, hda6, hda6ros1-4, drm1drm2cmt3(ddc),drm1drm2cmt3ros1-4(ddcros1-4). Values are means+s.d.’s per 25,000 μm2of 3-day-old cotyledon adaxial epidermis (n=3). Student’st-test, *P<0.01 (significantly different from Col). (h) Bisulfite sequencing analysis of theEPF2promoter, and (i) quantitative RT–PCR assay ofEPF2transcript levels in Col,ros1-4,nrpd1-3,nrpd1-3ros1-4, hda6andhda6ros1-4, drm1drm2cmt3(ddc),drm1drm2cmt3ros1-4(ddcros1-4). Student’st-test, *P<0.01 (significantly different fromros1-4). Error bars represent s.d.’s (n=4). (j) Small RNA northern blot analysis in Col,nrpd1-3,ros1-4andnrpd1-3ros1-4. tRNA and other RNA bands stained with ethidium bromide (EtBr) were used as loading control. miR167 was detected as an internal control. Arrows and arrowheads indicate the positions of size markers, 21 nt and 24 nt, respectively. Figure 5: Suppression of the ros1 epidermal patterning phenotype by RdDM mutations. ( a – f ) Adaxial epidermal cell phenotype of 3-day-old seedlings. ( a ) nrpd1-3 , ( b ) nrpd1-3ros1-4 , ( c ) hda6 , ( d ) hda6ros1-4 , ( e ) drm1-2drm2-2cmt3-13 ( ddc ) and ( f ) drm1-2drm2-2cmt3-13ros1-4 ( ddcros1-4 ). Images in a – f are at the same magnification. Scale bar, 30 μm. ( g ) Numbers of clustered small cells and stomata for Col, ros1-4, nrpd1-3, nrpd1-3ros1-4, hda6, hda6ros1-4, drm1drm2cmt3 ( ddc ), drm1drm2cmt3ros1-4 ( ddcros1-4 ). Values are means+s.d.’s per 25,000 μm 2 of 3-day-old cotyledon adaxial epidermis ( n =3). Student’s t -test, * P <0.01 (significantly different from Col). ( h ) Bisulfite sequencing analysis of the EPF2 promoter, and ( i ) quantitative RT–PCR assay of EPF2 transcript levels in Col, ros1-4 , nrpd1-3 , nrpd1-3ros1-4, hda6 and hda6ros1-4, drm1drm2cmt3 ( ddc ), drm1drm2cmt3ros1-4 ( ddcros1-4 ). Student’s t -test, * P <0.01 (significantly different from ros1-4 ). Error bars represent s.d.’s ( n =4). ( j ) Small RNA northern blot analysis in Col, nrpd1-3 , ros1-4 and nrpd1-3ros1-4 . tRNA and other RNA bands stained with ethidium bromide (EtBr) were used as loading control. miR167 was detected as an internal control. Arrows and arrowheads indicate the positions of size markers, 21 nt and 24 nt, respectively. Full size image In this study, we have provided strong evidence that ROS1-initiated active DNA demethylation is necessary for the expression of the EPF2 gene. Owing to the insertion of a hAT-like TE in the upstream region of EPF2 promoter, DNA methylation tends to spread from the TE into EPF2 promoter to cause silencing of EPF2 . ROS1 ensures EPF2 expression by erasing DNA methylation to control a proper population of stomatal lineage cells ( Fig. 6a,b ). The DNA methylation of the EPF2 promoter and silencing of EPF2 are dependent on RdDM. Our results suggest that ROS1 opposes RdDM action to ensure EPF2 expression ( Fig. 6c ). It was reported recently that low relative humidity triggers the methylation of SPCH and FAMA via RdDM [19] , [20] . It would be interesting to determine whether ROS1 may play a role in opposing the RdDM action on SPCH and FAMA under low humidity. It would also be interesting to investigate whether ROS1 function may be regulated by environmental and/or developmental cues. DME , another member of the ROS1 family of 5-methylcytosine DNA glycosylases/lyases [13] , is regulated by developmental cues since it is preferentially expressed in the central cell of the female gametophyte and in the progenitor of the endosperm [21] . The DME -mediated demethylation is necessary for genomic imprinting of the maternal allele of MEDEA and other genes in the endosperm [21] , [22] , [23] . DME is also important for the genomic demethylation in vegetative nuclei of developing pollens [24] , [25] , [26] . DME-mediated demethylation affects genes targeted by RdDM [27] , [28] . Initiation and maintenance of stem cell populations are important in all higher eukaryotes. Our study demonstrates that ROS1-initiated active DNA demethylation ensures the expression of EPF2 , and thereby is important for the size of the stomatal stem cell population in the leaf epidermis. Future research will determine whether active DNA demethylation may also be important for other stem cells in plants. 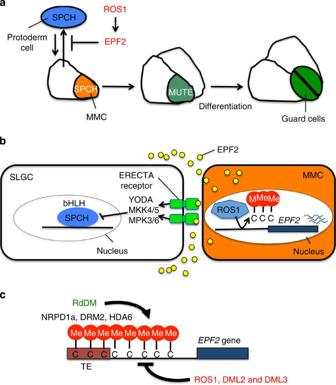Figure 6: A diagrammatic model of ROS1 function in stomatal development. (a) A model for ROS1 function in stomatal development. ROS1 negatively regulates the entry into the stomatal lineage throughEPF2. The bHLH protein SPCH is necessary for establishing the stomatal lineage. The bHLH protein MUTE is required for the termination of meristemoid asymmetric division and for the promotion of the GMC cell-state transition. (b) ROS1 removes DNA methylation from theEPF2promoter to enable expression of theEPF2gene, and EPF2 peptides are secreted outside of the meristemoid mother cell (MMC) to be received by the ERECTA receptor in the cell membranes of neighbour cells, stomatal lineage ground cell (SLGC). (c) ROS1 and RdDM antagonistically regulate the DNA methylation status of theEPF2promoter. Figure 6: A diagrammatic model of ROS1 function in stomatal development. ( a ) A model for ROS1 function in stomatal development. ROS1 negatively regulates the entry into the stomatal lineage through EPF2 . The bHLH protein SPCH is necessary for establishing the stomatal lineage. The bHLH protein MUTE is required for the termination of meristemoid asymmetric division and for the promotion of the GMC cell-state transition. ( b ) ROS1 removes DNA methylation from the EPF2 promoter to enable expression of the EPF2 gene, and EPF2 peptides are secreted outside of the meristemoid mother cell (MMC) to be received by the ERECTA receptor in the cell membranes of neighbour cells, stomatal lineage ground cell (SLGC). ( c ) ROS1 and RdDM antagonistically regulate the DNA methylation status of the EPF2 promoter. Full size image Plant materials The following mutants and transgenic lines were described previously: SPCHpro:nucGFP [3] , MUTEpro:nucGFP [29] , drm1-2drm2-2cmt3-11 ( ddc ) [30] , epf2-1 (ref. 6 ) (SALK_102777), spch-3 (ref. 3 ) (SAIL_36_B06), nrpd1-3 (SALK_128428) rdd [11] . rdd-2 is a triple mutant of ros1-4 (SALK_ 045303), dml2-2 (SALK_113573) and dml3-2 (SALK_056440). Arabidopsis T-DNA insertion lines were obtained from the Arabidopsis Biological Resource Center ( http://www.arabidopsis.org ). The hda6 mutant was kindly provided by Dr Zhizhong Gong (China Agricultural University). Construction of plasmid DNA EPF2 (CDS) was inserted into the cloning vector pTA7002 for inducible expression [31] . ROS1pro:ROS1 was inserted into the cloning vector pEARLEY GATE 301 (ref. 32 ) for ROS1 complementation analysis. Bisulfite sequencing One hundred nanograms of total DNA were analysed by sodium bisulfite genomic sequencing using the BisulFlash DNA Modification Kit (Epigentek; http://www.epigentek.com/catalog/index.php ) according to the manufacturer’s protocol. A 1-μl aliquot of bisulfite-treated DNA was used for each PCR reaction. PCR was performed in a total volume of 20 μl using ExTaq (Takara; http://www.takarabiousa.com/ ). Sequenced fragments were amplified with primers specific for each region ( Supplementary Table 1 ). Amplified PCR products were subcloned into the pCRII-TOPO vector (Invitrogen; http://www.invitrogen.com/site/us/en/home.html ) following the supplier’s instructions. For each region, more than 20 independent clones were sequenced from each sample. Microscopic observations Expanding cotyledons were stained with FM1-43 (Invitrogen; T35356), and fluorescence was detected with an Olympus BX53 fluorescence microscope with a GFP filter. A Leica SP5 confocal microscope was used for observation of GFP and FM4-64 (Invitrogen; F34653). Imaging conditions were excitation at 488 nm and a collecting bandwidth at 500–540 nm for GFP, and excitation at 561 nm and a collecting bandwidth at 600–645 nm for FM4-64. Small RNA northern blotting Total RNA was extracted from 2 g of 10-day-old seedlings, and the small RNA was enriched by PEG precipitation. A 30-μg quantity of small RNA per lane was run on a 15% acrylamide gel and then transferred to Hybond-N+ membranes. Hybridization followed the manufacturer’s instructions. DNA methylome data DNA methylome data (GEO accession GSE33071 ) were described previously [10] . How to cite this article: Yamamuro, C. et al . Overproduction of stomatal lineage cells in Arabidopsis mutants defective in active DNA demethylation. Nat. Commun. 5:4062 doi: 10.1038/ncomms5062 (2014).